R-loops and nicks initiate DNA breakage and genome instability in non-growingEscherichia coli Double-stranded DNA ends, often from replication, drive genomic instability, yet their origin in non-replicating cells is unknown. Here we show that transcriptional RNA/DNA hybrids (R-loops) generate DNA ends that underlie stress-induced mutation and amplification. Depleting RNA/DNA hybrids with overproduced RNase HI reduces both genomic changes, indicating RNA/DNA hybrids as intermediates in both. An Mfd requirement and inhibition by translation implicate transcriptional R-loops. R-loops promote instability by generating DNA ends, shown by their dispensability when ends are provided by I- Sce I endonuclease. Both R-loops and single-stranded endonuclease TraI are required for end formation, visualized as foci of a fluorescent end-binding protein. The data suggest that R-loops prime replication forks that collapse at single-stranded nicks, producing ends that instigate genomic instability. The results illuminate how DNA ends form in non-replicating cells, identify R-loops as the earliest known mutation/amplification intermediate, and suggest that genomic instability during stress could be targeted to transcribed regions, accelerating adaptation. DNA double-strand breaks and ends (DSBs/DSEs) are the single most potent inducers of genomic instability in cells from bacteria to human. Imperfectly accurate repair of DSBs/DSEs causes genomic rearrangements and small mutations that underlie breast [1] and other cancers [2] , many human genetic diseases [3] , evolution of pathogenic bacterial biofilms [4] , mutations that cause bacterial antibiotic resistance [5] , bacterial evasion of host defenses [6] , and stress-induced mutations (SIMs) that may accelerate evolution preferentially when cells are maladapted to their environments [7] , [8] , [9] . Although DNA breaks result from exogenous DNA-damaging agents, endogenous or spontaneous DSBs/DSEs are thought to be the commonest instigators of genomic instability mechanisms in all cells (for example, Vilenchik and Knudson [10] ). However, despite their paramount importance to genomic instability that drives evolution and disease, and although their rates of formation are being quantified [11] , mechanisms of spontaneous DNA breakage are poorly understood. Some mechanisms that produce spontaneous DSBs/DSEs are associated with DNA replication. First, when replication forks encounter single-stranded (ssDNA) breaks in the DNA template, they can ‘collapse’ producing a single DSE [12] (illustrated Fig. 1e ). Second, paused replication forks can be cleaved by endonucleases that cleave recombination intermediates creating DSEs [13] , [14] . Third, when converging replication and transcription complexes collide ‘head on’ on DNA, DSBs/DSEs can result [15] , [16] , though the precise mechanism of breakage is not known [17] . Fourth, DSBs/DSEs also result from co-directional collisions of the replisome with RNA polymerase (RNAP), when RNAP has ‘back-tracked’ on the DNA template [17] , [18] . DSEs produced by co-directional collisions are prevented by Mfd helicase, which dislodges the back-tracked RNAP [18] . Formation of these DSEs requires an RNA/DNA hybrid [18] and appears to result from the DNA polymerase stopping at the RNA/DNA hybrid ‘under’ the back-tracked RNAP. This leaves a ssDNA nick or gap in the new DNA strand [18] , [19] , which then becomes a DSE by fork collapse when a second round of replication encounters the nick (per Fig. 1e ). Thus, DSEs generated by co-directional collisions of the replisome with RNAP are: (1) prevented by Mfd helicase, and (2) caused by RNA/DNA hybrids plus replication. 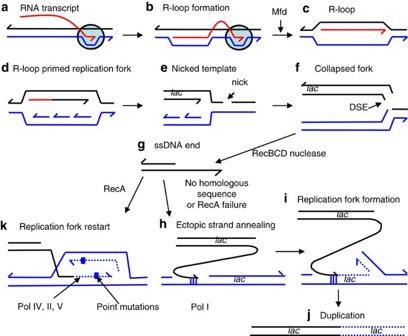Figure 1: Model for transcription-promoted R-loop initiation of DSEs. (a–c) R-loops form by incorporation of the transcript (red) into supercoiled DNA (blue/black) behind the site of transcription41. R-loop formation is usually inhibited by ribosomes or the R-loop removed by RNase HI. (b) Stalled RNAP (circle) (c) is removed by Mfd38. (d) The R-loop can then form a replication fork35. (e) If the replication fork encounters a nick in a template DNA strand, the fork will collapse (f), forming a single DSE12. In stressed cells, the collapsed fork might be repaired and restarted by microhomology-mediated break-induced replication (g–j)26producing genome rearrangements (duplication shown here). (g) DSE degradation and 5′-end resection by RecBCD might be followed byhannealing of the overhanging 3′-end to ssDNA at a site of microhomology (vertical lines), shown here in the lagging-strand template of another replication fork (blue). (i,j) This replication restart is shown at a position behind where the initial fork collapsed, so that a segment of the genome including thelacregion becomes duplicated. The duplication can be expanded into an amplified array by unequal crossing-over (not illustrated). (k) Alternatively, point mutation is proposed to occur when the DSE is repaired by homologous recombination-mediated replication-fork restart using error-prone polymerase Pol IV during restart due to licensing of Pol IV (and also Pols II and V) by the RpoS and SOS stress responses9,21,24. Figure 1: Model for transcription-promoted R-loop initiation of DSEs. ( a – c ) R-loops form by incorporation of the transcript (red) into supercoiled DNA (blue/black) behind the site of transcription [41] . R-loop formation is usually inhibited by ribosomes or the R-loop removed by RNase HI. ( b ) Stalled RNAP (circle) ( c ) is removed by Mfd [38] . ( d ) The R-loop can then form a replication fork [35] . ( e ) If the replication fork encounters a nick in a template DNA strand, the fork will collapse ( f ), forming a single DSE [12] . In stressed cells, the collapsed fork might be repaired and restarted by microhomology-mediated break-induced replication ( g – j ) [26] producing genome rearrangements (duplication shown here). ( g ) DSE degradation and 5′-end resection by RecBCD might be followed by h annealing of the overhanging 3′-end to ssDNA at a site of microhomology (vertical lines), shown here in the lagging-strand template of another replication fork (blue). ( i , j ) This replication restart is shown at a position behind where the initial fork collapsed, so that a segment of the genome including the lac region becomes duplicated. The duplication can be expanded into an amplified array by unequal crossing-over (not illustrated). ( k ) Alternatively, point mutation is proposed to occur when the DSE is repaired by homologous recombination-mediated replication-fork restart using error-prone polymerase Pol IV during restart due to licensing of Pol IV (and also Pols II and V) by the RpoS and SOS stress responses [9] , [21] , [24] . Full size image Whereas the mechanisms of DSB/DSE generation listed above require replicating DNA, DSBs/DSEs also provoke SIM pathways in starvation-stressed cells that are unlikely to be replicating DNA. DSBs/DSEs initiate two mechanisms of SIM in starving Escherichia coli cells: stress-induced point mutation [9] , [20] , [21] and gene amplification [21] , [22] (reviewed in refs 7 , 8 , 9 ). Both mechanisms occur via repair of DSBs/DSEs that becomes mutagenic upon activation of the RpoS-controlled general stress response [23] . The point mutation mechanism is an RpoS-controlled switch to mutagenic DSE repair in which replication primed from DSEs uses error-prone DNA polymerases when RpoS is activated, causing indel and base-substitution mutations [9] , [21] , [24] , [25] (illustrated Fig. 1g ). The amplification mechanism causes genome rearrangements [22] , [26] , [27] (reviewed in Hastings et al . [28] ) is also thought to result from DSE-initiated replication [21] , [22] ( Fig. 1g–j ) and requires RpoS [23] . Thus, parts g–k of Fig. 1 represent current understanding based on much previous work. Stress-induced point mutation occurs both in a Lac plasmid-based mutation assay [29] and in chromosomes of plasmid-free cells [9] , [24] , [25] , [30] , and underlies half of spontaneous base-substitution and frameshift mutagenesis in the chromosomes of starving E. coli [24] , and so is likely to be important to evolution. Amplification is an important model for mechanisms of human copy-number variation [28] . The origin of DSBs/DSEs in non-replicating cells, including the DSEs that that underlie SIM, is poorly understood. At sites in an F′ plasmid, SIM requires TraI ssDNA endonuclease [21] , which makes ssDNA nicks in the F plasmid. As TraI is not needed when DSBs are delivered to the F using double-stranded endonuclease I- Sce I, ssDNA nicks are inferred to promote SIM by causing DSB/DSEs [21] , for example via fork collapse ( Fig. 1e ). Cells that express a phage ssDNA endonuclease and carry its cleavage site in the F′ do not require TraI for point mutation, implying that any ssDNA nick will allow SIM [31] . However, spontaneous DSBs/DSEs also promote mutation in starving plasmid-free E. coli [9] , [24] , indicating that DSBs/DSEs also form independently of TraI. Given that replication is repressed during starvation, that at least some of the SIM-promoting DSEs probably arise from fork collapses [21] , [31] , [32] , and that most models for the origins of spontaneous DSEs involve replication, how spontaneous DSEs form in starvation-stressed non-growing cells is unclear. If fork collapse is the mechanism, then how and where do the forks originate? If not, then how are the ssDNA nicks converted into the DSEs that underlie SIM? How spontaneous DSEs are formed in non-replicating cells, and how replication-dependent processes (for example, Fig. 1 ) can occur in starved, non-replicating cells are important and fundamental problems, the solution to which is likely to pertain to many different organisms and circumstances. DNA replication in growing cells is initiated at fixed sites (origins). Origin activity is repressed in stationary-phase cells [33] . However, origin-independent replication can be initiated by RNA paired with unbroken DNA (R-loops, Fig. 1c ) and at D-loops (similar structures made solely of DNA) under some circumstances [34] , [35] . Here, we provide evidence that DSE production is promoted by R-loops in starving cells. We show that RNA/DNA hybrids produced by transcription (R-loops) are precursors to the DSBs/DSEs that initiate stress-induced amplification (genome rearrangement) and point mutation, making R-loops the earliest known molecular intermediate for both processes. We show that R-loops provoke DSBs/DSEs by a two-step mechanism that is unlike the co-directional collision mechanism. We suggest that R-loop-primed replication forks collapse at independent ssDNA nicks to generate DSEs ( Fig. 1a–f ). This mechanism may explain DSE formation in many circumstances, particularly in non-replicating cells in which firing of standard replication origins is suppressed. RNA/DNA hybrids underlie stress-induced genomic changes We used the E. coli Lac assay for stress-induced point mutation [29] and gene amplification [36] . In this assay, cells carrying a lac +1 bp frameshift allele in an F′ plasmid are grown to saturation in liquid, then spread on solid lactose minimal medium on which they starve. Lac + revertant colonies are of three types (for example, Fig. 2a ): generation-dependent mutants that occurred during the liquid growth of the culture before starvation on lactose appear as colonies on day 2 (ref. 29 ); and stress-induced point-mutant and lac- amplified clones, formation of which requires activation of the RpoS stress response [23] , are visible as Lac + colonies from day 3 onward. Point mutants dominate early (for example, Fig. 2a ), and amplified clones rise from ~5% of Lac + colonies on day 5 to ~40% by day 8 (ref. 36 ). Point-mutant and amplified colonies are distinguished by appearance on color-indicator medium (Methods). 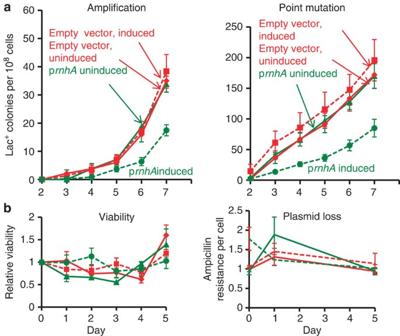Figure 2: Overproduction of RNase HI reduces stress-induced amplification and point mutation. (a) Gene amplification and point mutation in strain PJH1093, carrying prnhA(pBAD18-rnhA). Production of RNase HI is uninduced () (solid line) or induced () (broken line) by the presence of arabinose. Also strain PJH1091, carries empty vector pBAD18 as a control, with transcription from the PBADpromoter induced (♦) or uninduced () by presence or absence of arabinose respectively. (b) Viability and retention of pBAD18-rnhAby day 5 of the experiment shows no plasmid loss. Viability and plasmid loss plots are offset by 2 days: the time needed to form a visible Lac+colony. Error bars, one s.e.m. of four parallel cultures. These and all experiments were performed three times with comparable results. Figure 2: Overproduction of RNase HI reduces stress-induced amplification and point mutation. ( a ) Gene amplification and point mutation in strain PJH1093, carrying p rnhA (pBAD18- rnhA ). Production of RNase HI is uninduced ( ) (solid line) or induced ( ) (broken line) by the presence of arabinose. Also strain PJH1091, carries empty vector pBAD18 as a control, with transcription from the P BAD promoter induced (♦) or uninduced ( ) by presence or absence of arabinose respectively. ( b ) Viability and retention of pBAD18- rnhA by day 5 of the experiment shows no plasmid loss. Viability and plasmid loss plots are offset by 2 days: the time needed to form a visible Lac + colony. Error bars, one s.e.m. of four parallel cultures. These and all experiments were performed three times with comparable results. Full size image We find that overproduction of RNase HI, which degrades the RNA from RNA/DNA hybrids [37] , reduces stress-induced amplification and point mutation ( Fig. 2a ). Preliminary experiments showed that overproduction of RNase HI, encoded by rnhA , from the arabinose-inducible P BAD promoter in plasmid pBAD18 -rnhA , inhibits growth. We used the highest concentration of arabinose that did not inhibit growth of cells containing this plasmid (5 × 10 −8 (w/v)). Overproduction of RNase HI-reduced amplification and point mutation to about 60% (representative experiments, Fig. 2a ), presumably by reducing levels of RNA/DNA hybrids. In three experiments, amplification was reduced to 56±8%, days 2–7 ( P =0.017, Student’s t -test). For point mutation, the decrease was to 57±14%, days 2 to 7, ( P =0.047, Student’s t -test). There was no loss of pBAD18- rnhA or loss of cell viability during the experiment ( Fig. 2b ). Amplification and point mutation rates were unaffected by the empty vector with or without arabinose, and were the same as in cells uninduced for pBAD18- rnhA ( Fig. 2a ). These data imply that about half of amplification and point mutagenesis requires an RNA/DNA hybrid intermediate, and that removal of the RNA/DNA hybrid by overproduced RNase HI curtails both processes. Loss of RNase HI increases amplification and mutation We find that knock out of RNase HI increases both amplification and point mutation ~3-fold ( Fig. 3 ). In three experiments, amplification was increased by 2.9±0.01-fold, days 2–7 ( P =0.003, Student’s t -test), and point mutation by 3.1±0.3-fold, days 2–5, ( P =0.006, Student’s t -test). Thus, failure to remove RNA/DNA hybrids promotes both processes. Cell viability was unaffected. These data support the conclusion that RNA/DNA hybrids promote both amplification and point mutation. 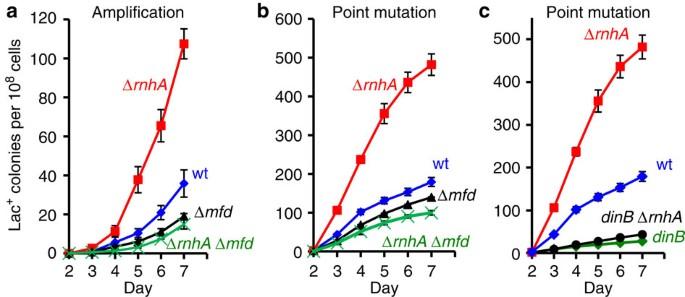Figure 3: Loss of RNase HI increases amplification and point mutation. (a,b) Mfd is required for approximately half of amplification and point mutation inrnhA+(‘wild-type’) cells and all the increase in point mutation and amplification in RNase HI-defective (ΔrnhA) cells. Gene amplification and point mutation in (a) and (b); wild-type (♦), ΔrnhA(),mfd(), andmfdΔrnhA( × ) strains SMR4562, PJH683, PJH813 and PJH946. (c) Increased point mutation in cells lacking RNase HI requires DinB/DNA Pol IV, as in RNase HI-proficient cells43. Wild-type (♦), ΔrnhA(),dinB10(♦),dinB10ΔrnhA() strains SMR4562, PJH683, SMR5830 and PJH791. Error bars, one s.e.m. of four parallel cultures. These experiments were performed three times with comparable results. Figure 3: Loss of RNase HI increases amplification and point mutation. ( a , b ) Mfd is required for approximately half of amplification and point mutation in rnhA + (‘wild-type’) cells and all the increase in point mutation and amplification in RNase HI-defective (ΔrnhA) cells. Gene amplification and point mutation in ( a ) and ( b ); wild-type (♦), Δ rnhA ( ), mfd ( ), and mfd Δ rnhA ( × ) strains SMR4562, PJH683, PJH813 and PJH946. ( c ) Increased point mutation in cells lacking RNase HI requires DinB/DNA Pol IV, as in RNase HI-proficient cells [43] . Wild-type (♦), Δ rnhA ( ), dinB10 (♦), dinB10 Δ rnhA ( ) strains SMR4562, PJH683, SMR5830 and PJH791. Error bars, one s.e.m. of four parallel cultures. These experiments were performed three times with comparable results. Full size image Instability promoted by RNA/DNA hybrids requires Mfd Mfd helicase is a transcription accessory protein that associates with RNAP [38] , couples nucleotide-excision repair to transcription in transcription-coupled repair [39] , and, when a replication folk collides with active RNAP, mediates the conflict by removing RNAP [40] . Mfd prevents the formation of DSBs/DSEs caused by co-directional collisions of the replisome with RNAP [18] . By removing stalled RNAP, Mfd also frees the 3′-terminus of the nascent transcript. Processes affected by Mfd are inferred to involve transcription. We find that the increased amplification and point mutation seen in RNase HI-defective strains requires Mfd (representative experiment, Fig. 3a ). This indicates that the RNA/DNA hybrids that promote amplification and mutation arise from transcription, and are in the form of R-loops. Knock out of Mfd also decreases amplification in RNase HI-proficient cells to about half ( Fig. 3a ). In three experiments, amplification was reduced to 0.63±0.08, days 2–7 ( P =0.023, Student’s t -test). For point mutation, the decrease was less, but significant (0.75±0.02-fold, days 2–7, P =0.002, Student’s t -test). This result resembles the two-fold reduction of amplification and point mutation by overproduction of RNase HI ( Fig. 2a ), implying that Mfd also promotes those R-loop-instigated genomic changes. These data support the conclusion that at least half of mutagenesis and amplification in wild-type cells proceeds through RNA/DNA hybrid intermediates and that these intermediates are R-loops at sites of transcription. Translation inhibition increases instability Formation of transcriptional R-loops in bacteria is inhibited by ribosomes on the nascent transcript [41] such that inhibiting protein synthesis increases levels of transcription-generated R-loops. We find that pulse-inhibition of ribosome progression increases amplification and point mutation ( Fig. 4 ), supporting the hypothesis that both are promoted by transcriptional R-loops. We treated stationary-phase cultures with spectinomycin, an inhibitor of ribosome translocation [42] , for 3 h before plating on lactose medium and observed a ~2-fold increase in amplification (2.2±0.4-fold, three experiments, P =0.048, Student’s t -test). Point mutation increased less but still significantly (1.23±0.06-fold, three experiments, P =0.024, Student’s t -test) ( Fig. 4a ). These increases require Mfd ( Fig. 4a ), supporting the transcriptional origin of the spectinomycin-induced increases. The increased point mutation caused by translational inhibition ( Fig. 4c ) and loss of RNase HI ( Fig. 3c ) both require DinB/Pol IV, indicating that it occurs by the usual Pol IV-dependent [43] pathway. 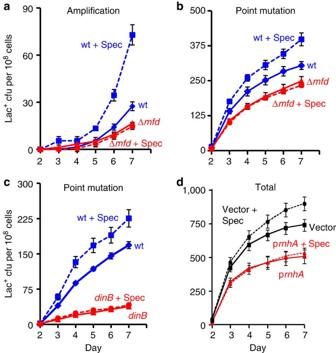Figure 4: Inhibition of translation increases amplification and point mutation. Gene amplification (a) and point mutation (b) in WT (SMR4562) andmfd(PJH813) strains pulsed with spectinomycin (spec) (broken lines). WT+spec (), WT (♦),mfd+spec (),mfd(). (c) The spectinomycin treatment-induced increase in point mutagenesis is DinB/Pol IV-dependent. Point mutation in WT (SMR4562) anddinB(SMR5830) cells pulsed with spec. WT+spec (), WT (♦),dinB+spec (),dinB(). The curves for the spectinomycin-treated WT cells differ from those of the untreated WT cells significantly, WT and spec-treated WT differ (for three experiments,P=0.002 for point mutation and 0.001 for amplification, Student’st-test);mfdand spec-treatedmfdare not significantly different (P=0.6 for point mutation, and 0.7 for amplification). (d) Spectinomycin treatment does not increase Lac+revertants in cells overproducing RNase HI. Vector pBAD18 (), vector pBAD18 spec-treated (), pBAD18-rnhA(), pBAD18-rnhAspec-treated (); broken lines denote spectinomycin treatment. Error bars represent one s.e.m. of four parallel cultures. These experiments were performed three times with comparable results. Figure 4: Inhibition of translation increases amplification and point mutation. Gene amplification ( a ) and point mutation ( b ) in WT (SMR4562) and mfd (PJH813) strains pulsed with spectinomycin (spec) (broken lines). WT+spec ( ), WT (♦), mfd +spec ( ), mfd ( ). ( c ) The spectinomycin treatment-induced increase in point mutagenesis is DinB/Pol IV-dependent. Point mutation in WT (SMR4562) and dinB (SMR5830) cells pulsed with spec. WT+spec ( ), WT (♦), dinB +spec ( ), dinB ( ). The curves for the spectinomycin-treated WT cells differ from those of the untreated WT cells significantly, WT and spec-treated WT differ (for three experiments, P =0.002 for point mutation and 0.001 for amplification, Student’s t -test); mfd and spec-treated mfd are not significantly different ( P =0.6 for point mutation, and 0.7 for amplification). ( d ) Spectinomycin treatment does not increase Lac + revertants in cells overproducing RNase HI. Vector pBAD18 ( ), vector pBAD18 spec-treated ( ), pBAD18- rnhA ( ), pBAD18- rnhA spec-treated ( ); broken lines denote spectinomycin treatment. Error bars represent one s.e.m. of four parallel cultures. These experiments were performed three times with comparable results. Full size image Supporting the hypothesis that spectinomycin increases mutation by increasing R-loop formation, we find that overproduction of RNase HI suppresses spectinomycin-enhanced mutagenesis ( Fig. 4d ). Spectinomycin increased mutation in the control-plasmid-carrying strain 1.34±0.09-fold (mean±s.e.m. of four experiments) but not the RNase HI-overproducing strain ( Fig. 4d ), which, with or without spectinomycin treatment, showed 0.58±0.23 of the level of mutation in the untreated control-plasmid strain ( Fig. 4d , mean±s.e.m. of four experiments). We conclude that the mutation-promoting effect of spectinomycin is prevented by removal of RNA/DNA hybrids. Although inhibition of translation might affect cells in various ways, both the Mfd-dependence ( Fig. 4a ) and the dependence on RNA/DNA hybrids ( Fig. 4d ) support the interpretation that translation inhibition promotes amplification and mutagenesis by stabilizing transcriptional R-loops. Endonuclease-induced breaks substitute for R-loops In principle, R-loops might promote SIM by promoting DSB/DSEs ( Fig. 1b–f ) or by promoting some stage of the SIM mechanisms downstream of DSE formation ( Fig. 1g–k ). Stress-induced point mutation and amplification mechanisms can be separated experimentally into the stages that occur before or after formation of DSEs ( Fig. 1g–k , reviewed in Rosenberg et al . [9] and Hastings et al . [28] ). Proteins or DNA intermediates that promote SIM because they promote DSE formation are not required if DSBs are created near lac with I- Sce I site-specific endonuclease [21] , as shown for TraI ssDNA endonuclease [21] and the major role of the σ E response [44] . By contrast, proteins that promote SIM at stages after creation of DSEs remain required when DSBs are provided by I- Sce I (near lac [21] , or near chromosomal mutation-reporter genes [24] , [25] , [30] ). We used I- Sce I to address whether R-loops promote SIM by acting before or after DSE creation. Although I- Sce I decreases viability, the RNase HI plasmid does not ( Fig. 5c ), allowing us to compare the rates of Lac reversion with and without the RNase HI plasmid. 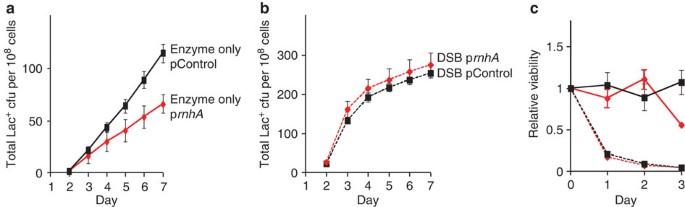Figure 5: R-loops are not needed for mutagenesis when DSBs are caused by I-SceI. Overproduction of RNase HI (reduction in R-loops) does not decrease mutagenesis when I-SceI-generated DSBs are provided. (a) The RNase HI-overproducing strain (PJH1239) (♦) shows about half as much Lac+mutation as the strain carrying the control plasmid (PJH1237) (). (b) The DSB-producing strain (carrying the chromosomal inducible I-SceI enzyme and I-SceI cutsite nearlac) that over-produces RNase HI (PJH1321) (♦) shows no reduction of Lac+mutants compared with the isogenic strain carrying the control plasmid (PJH1319) (), indicating that R-loops are not necessary for mutation when DSBs are provided. This result holds when both I-SceI enzyme and cutsite are present and not in strains with the enzyme only (a). (c) Strains experiencing double-strand cutting by I-SceI show reduced viability. However, the viability decrease is the same for cells with thernhAplasmid as for those with the control plasmid making quantitative comparisons meaningful. Relative viability was determined per21. Values in (a,b) have not been corrected for declining viability. Error bars represent one s.e.m. of four parallel cultures. Each experiment was performed three times with comparable results. Figure 5: R-loops are not needed for mutagenesis when DSBs are caused by I- Sce I. Overproduction of RNase HI (reduction in R-loops) does not decrease mutagenesis when I- Sce I-generated DSBs are provided. ( a ) The RNase HI-overproducing strain (PJH1239) (♦) shows about half as much Lac + mutation as the strain carrying the control plasmid (PJH1237) ( ). ( b ) The DSB-producing strain (carrying the chromosomal inducible I- Sce I enzyme and I- Sce I cutsite near lac ) that over-produces RNase HI (PJH1321) (♦) shows no reduction of Lac + mutants compared with the isogenic strain carrying the control plasmid (PJH1319) ( ), indicating that R-loops are not necessary for mutation when DSBs are provided. This result holds when both I- Sce I enzyme and cutsite are present and not in strains with the enzyme only ( a ). ( c ) Strains experiencing double-strand cutting by I- Sce I show reduced viability. However, the viability decrease is the same for cells with the rnhA plasmid as for those with the control plasmid making quantitative comparisons meaningful. Relative viability was determined per [21] . Values in ( a , b ) have not been corrected for declining viability. Error bars represent one s.e.m. of four parallel cultures. Each experiment was performed three times with comparable results. Full size image Figure 5b shows that when DSBs are made by I- Sce I, Lac + reversion is unaffected by overproduction of RNase HI. This contrasts with reduction of Lac reversion caused by RNase HI overproduction in cells without I- Sce I-induced DSBs, either when no I- Sce I is present ( Fig. 2a ) or in the presence of the I- Sce I enzyme but no cutsite ( Fig. 5a ). We conclude that R-loops become superfluous for mutagenesis when a DSB is provided independently. In three experiments, in the absence of I- Sce I cutting (‘enzyme-only’ control), RNase HI overproduction reduced the Lac + reversion rate by a significant 1.7±0.2-fold (mean±s.e.m.) relative to the control plasmid (Lac + colonies per day, day 3 to day 5). In contrast, when DSBs were induced, RNase HI overproduction caused 1.23±0.06 times more Lac + reversion than seen with the control plasmid. The lack of effect of RNase H overproduction in strains with I -Sce I cuts is significantly different from its effect without I- Sce I ( P =0.013, Student’s t -test). We conclude that R-loops contribute to DSB or DSE generation and so are not needed if DSBs are provided. We could not distinguish amplification from point mutation in these experiments because of the low proportion of lac -amplified colonies. lac -amplified colonies appear later than point mutants [36] , and so are more affected by loss of viability over time. Also, although amplification is stimulated by I- Sce I cuts made near lac , point mutation is stimulated more than amplification [21] , because co-amplification of the cutsite with lac causes loss of the repeats [21] . These results indicate that R-loops function in the mutagenesis pathway upstream of (leading to the production of) the DSBs or DSEs that initiate mutagenesis. Formation of R-loop-promoted DSEs requires a ssDNA nick In this section and the next, we provide two additional, independent lines of support for the conclusion that R-loops promote SIM by creation of DSEs. We also show that they do so in a two-step process that additionally requires a ssDNA nick. First, we produced the DSE-binding Gam protein from phage Mu in RNase HI-deletion cells. Gam binds to DSEs and prevents them from being processed by nucleases [45] , and thus prevents DSE-induced recombination [46] . We produced Gam from the chromosome controlled by a doxycycline-inducible promoter. Doxycycline induction of Gam reduces amplification and point mutation ( Fig. 6 ), confirming that both mechanisms require a DSE that is blocked by Gam. Importantly, induction of Gam prevents the increase of amplification and point mutation seen otherwise in RNase HI-defective cells, in which R-loops accumulate. These results show that the SIM promoted by R-loops in RNase HI-defective cells requires DSEs, and does not result from a different, DSE-independent pathway. 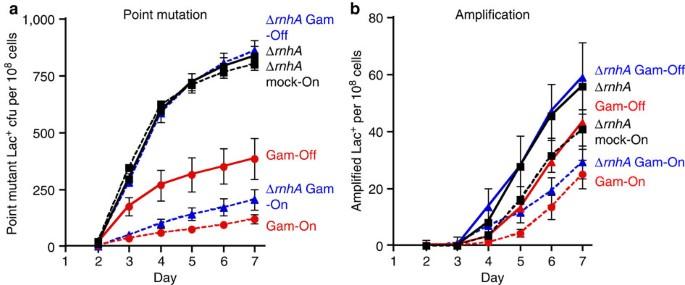Figure 6: Gam prevents R-loops from initiating amplification and point mutation. The increased amplification and mutation seen in cells with increased R-loops due to knock out of RNase HI (ΔrnhA) is prevented by doxycycline-induced production of Gam protein (Gam-On) (Methods). Gam binds DSEs45, prevents them engaging in repair46and reduces (a) point mutation and (b) amplification, confirming that DSEs are required for both pathways. Doxycycline-induced production of Gam protein (Gam-On) prevents the increase inapoint mutation andbamplification caused by knock out of RNase HI (ΔrnhA), demonstrating that the increased R-loops cause increased amplification and point mutation via DSEs. Strains: ΔrnhA tetRPJH2039 (); ΔrnhA PN25tetOgam tetR, PJH2443 ();PN25tetOgam tetR, PJH2023 ().Gam-On induction, broken lines. Gam-Off, the same strains as ‘Gam-On’ without doxycycline induction; mock-On, strains with the Tet repressor but without thegamgene treated with doxycycline. Error bars represent one s.e.m. of four parallel cultures. This experiment was performed three times with comparable results. Figure 6: Gam prevents R-loops from initiating amplification and point mutation. The increased amplification and mutation seen in cells with increased R-loops due to knock out of RNase HI (Δ rnhA ) is prevented by doxycycline-induced production of Gam protein (Gam-On) (Methods). Gam binds DSEs [45] , prevents them engaging in repair [46] and reduces ( a ) point mutation and ( b ) amplification, confirming that DSEs are required for both pathways. Doxycycline-induced production of Gam protein (Gam-On) prevents the increase in a point mutation and b amplification caused by knock out of RNase HI (Δ rnhA ), demonstrating that the increased R-loops cause increased amplification and point mutation via DSEs. Strains: Δ rnhA tetR PJH2039 ( ); Δ rnhA P N25tetO gam tetR , PJH2443 ( ); P N25tetO gam tetR , PJH2023 ( ).Gam-On induction, broken lines. Gam-Off, the same strains as ‘Gam-On’ without doxycycline induction; mock-On, strains with the Tet repressor but without the gam gene treated with doxycycline. Error bars represent one s.e.m. of four parallel cultures. This experiment was performed three times with comparable results. Full size image Second, we suggest a two-step model in which R-loops generate DSEs in stationary cells by priming replication forks that become DSEs when they encounter a ssDNA nick ( Fig. 1a–f , Introduction). R-loops can prime replication independently of standard origins in RNase H-defective cells [34] , [35] and in solution with purified proteins [19] . In the F′ plasmid, ssDNA nicks are made constitutively by TraI, a site-specific ssDNA endonuclease that nicks the F′ transfer origin, and which is required for SIM at sites in the F′ [21] . The antimutagenic effect of deleting traI is more than suppressed by providing I- Sce I-generated DSEs near lac [21] , showing that TraI contributes to formation of DSEs that drive mutagenesis, presumably by fork collapse at the ssDNA nick ( Fig. 1e ) [7] , [21] . We suggest that R-loops cause DSEs by priming replication forks that collapse at a ssDNA nick ( Fig. 1a–f ). This model predicts that ssDNA nicks made by TraI will be required for the R-loop-mediated production of DSEs. Conversely, if R-loops promoted DSE formation independently of ssDNA nicks, we might find that although TraI is required for most mutagenesis in RNase HI + cells [21] , it would not be required for the extra mutagenesis observed in RNase HI-defective cells. Supporting the two-step R-loop-plus-ssDNA-nick model ( Fig. 1 ), Fig. 7 shows that most mutation induced in RNase HI knockout cells requires TraI. Whereas Δ traI reduced mutation rate in otherwise wild-type cells about 60-fold, it reduced the rate in RNase HI-defective cells 108-fold ( Fig. 7 , Supplementary Table S1 ), showing a very strong requirement for TraI in the mutagenesis promoted by R-loops. Thus, most DSEs generated by R-loops in the F′ form in a process that also requires the ssDNA nick made by TraI. 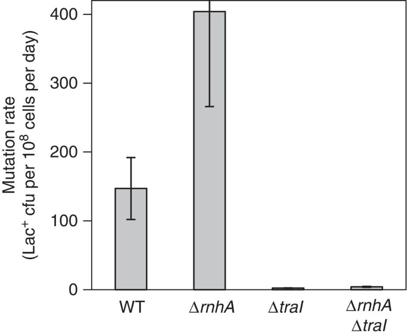Figure 7: R-loop-promoted mutagenesis requires ssDNA endonuclease TraI. The abundance of R-loops caused by deletion ofrnhAis not sufficient, but also requires TraI-generated ssDNA nicks, to promote mutagenesis. Therefore generation of DSEs by R-loops requires both an R-loop and a ssDNA nick. Strains: WT, SMR4562; ΔrnhA,PJH683; ΔtraI,PJH234; ΔrnhAΔtraI,PJH 963. Mean±s.e.m. of three experiments. Figure 7: R-loop-promoted mutagenesis requires ssDNA endonuclease TraI. The abundance of R-loops caused by deletion of rnhA is not sufficient, but also requires TraI-generated ssDNA nicks, to promote mutagenesis. Therefore generation of DSEs by R-loops requires both an R-loop and a ssDNA nick. Strains: WT, SMR4562; Δ rnhA, PJH683; Δ traI, PJH234; Δ rnhA Δ traI, PJH 963. Mean±s.e.m. of three experiments. Full size image A small fraction of the extra R-loop-promoted SIM in RNase HI null cells is TraI-independent, in that knock out of RNase HI increased mutation slightly but just significantly in TraI-defective cells (1.8-fold, mean of three experiments, P =0.0376, Student’s t -test). This could result from spontaneous ssDNA nicks ( Fig. 1a–f ). We conclude that ssDNA nicks are required for most of the mutagenesis promoted by R-loops. This supports the hypothesis that R-loops generate the breaks in these stationary cells via the two-step mechanism in which the RNA primes replication that collapses at a ssDNA nick producing a DSE ( Fig. 1a–f ). This is unlike DSEs generated by co-directional collisions in replicating cells, in which the R-loop itself is thought to create a ssDNA nick [18] . In molecules other than F, spontaneous ssDNA nicks, which are ubiquitous and common [47] , are expected to play this role. R-loops plus single-stranded nicks generate visible DSEs We used a visual assay to show directly that R-loops generate DSEs, and that DSE formation requires both the R-loop and a ssDNA nick. We assayed DSEs in living cells by quantifying cells with visible foci of the DSE-labelling GamGFP fusion protein (Methods) in the E. coli chromosome, and in the F′ plasmid in which amplification and point mutation were assayed. 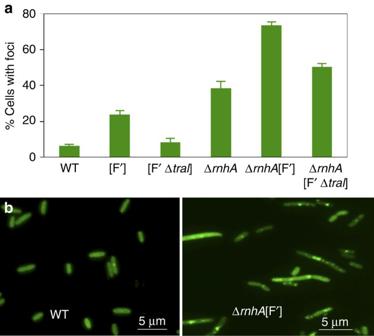Figure 8: Formation of DSEs promoted by R-loops also requires ssDNA nicks. (a) Quantification of cells with GamGFP foci. Cells carrying the F′ plasmid show more foci than F−(WT) cells, and these extra foci are TraI-dependent, and thus result from the ssDNA nicks made by TraI endonuclease atoriT.Cells lacking RNase HI show more foci than their isogenic RNase HI+parents (compare WT with ΔrnhA; and [F′] with ΔrnhA[F′]) indicating that lack of RNase HI (increased R-loops) causes increased DSEs. Finally, the increased foci caused by loss of RNase HI in the F′ (compared with that in F−ΔrnhAcells) requires TraI ssDNA endonuclease. Therefore, R-loop-mediated foci require both the R-loopanda ssDNA nick. Means±s.e.m. of three experiments. WT ‘wild-type’ SMR14015; [F′] SMR16387; [F′ΔtraI] SMR16475; ΔrnhASMR16379; ΔrnhA[F′] SMR16389; ΔrnhA[F′ΔtraI] SMR16477. All strains carry a chromosomaltetRand PN25tetOgam-gfp.Supplementary Table S2for numerical values. (b) Examples of fields of cells showing few GamGFP foci in wild-type, SMR14015, and multiple foci in most cells in ΔrnhA[F′], SMR16389. Figure 8b shows a representative example of the results, which are quantified in Fig. 8a and Supplementary Table S2 . The following points are evident ( Supplementary Table S2 , Fig. 8a ): first, 24% of cells with an F′ showed foci, whereas only 6.3% of F − cells did, indicating that the difference (17.7%) is foci caused by DSEs in the F′. Second, those F′-specific DSEs are mostly TraI-dependent, because they are reduced to 8% when TraI is deleted (the 6% in F − cells and 8% in cells with a TraI-defective F′ are not significantly different, P= 0.904, Student’s t -test). Third, knockout of RNase HI increased the number of F − and F′-carrying cells with foci to 38% (from 6.3% in WT) and 73% (from 24% in [F′]), respectively, showing that R-loops promote DSE formation robustly in both the chromosome and F′. Fourth, most GamGFP foci in RNase HI-defective cells with an F′ are TraI-dependent. Whereas 73±2% of F′ RNase HI-deletion cells show foci, only 50±2% of F′ RNase HI-deletion cells lacking TraI do. This number is not significantly higher than the 38±4% of F − RNase HI-deletion cells that show foci ( Supplementary Table S2 , Fig. 8a , P =0.07, Student’s t -test), suggesting that most of the increased DSBs caused by F are caused by TraI activity. Figure 8: Formation of DSEs promoted by R-loops also requires ssDNA nicks. ( a ) Quantification of cells with GamGFP foci. Cells carrying the F′ plasmid show more foci than F − (WT) cells, and these extra foci are TraI-dependent, and thus result from the ssDNA nicks made by TraI endonuclease at oriT. Cells lacking RNase HI show more foci than their isogenic RNase HI + parents (compare WT with Δ rnhA ; and [F′] with Δ rnhA [F′]) indicating that lack of RNase HI (increased R-loops) causes increased DSEs. Finally, the increased foci caused by loss of RNase HI in the F′ (compared with that in F − Δ rnhA cells) requires TraI ssDNA endonuclease. Therefore, R-loop-mediated foci require both the R-loop and a ssDNA nick. Means±s.e.m. of three experiments. WT ‘wild-type’ SMR14015; [F′] SMR16387; [F′Δ traI ] SMR16475; Δ rnhA SMR16379; Δ rnhA [F′] SMR16389; Δ rnhA [F′Δ traI ] SMR16477. All strains carry a chromosomal tetR and P N25tetO gam - gfp. Supplementary Table S2 for numerical values. ( b ) Examples of fields of cells showing few GamGFP foci in wild-type, SMR14015, and multiple foci in most cells in Δ rnhA [F′], SMR16389. Full size image Overall, the data confirm that first, DSEs, assayed directly as GamGFP foci, are promoted by R-loops, and second, that the R-loop-promoted DSE foci also require a second event, a ssDNA nick, which in the F′ is usually generated by TraI. This supports the two-step R-loop-plus-nick model in Fig. 1a–f , in which R-loops promote DSE formation by priming replication forks that collapse at a ssDNA nick. The results presented demonstrate a mechanism of generation of DSBs/DSEs by R-loops in starving, stationary-phase E. coli cells that requires Mfd translocase and also depends on ssDNA nicks. Because ssDNA nicks are common, spontaneously [47] this mechanism is likely to be generally important. We suggest that replication forks initiated from R-loops in stationary cells collapse, generating DSEs at independently occurring ssDNA nicks ( Fig. 1a–f ). This model can explain how DSEs can occur in non-replicating cells, in which standard origin-dependent replication is inhibited, in contrast with most current models for spontaneous DSE production (reviewed in the Introduction). R-loops were inferred previously to initiate replication in RNase HI- or RecG-defective cells [35] , and origin-independent replication (not demonstrably primed by R-loops) was seen in RNase HI + RecG + cells returned to growth upon entry to stationary phase [48] . This mechanism might be R-loop-independent and also does not resemble R-loop-promoted DNA breakage demonstrated here, in that it is RecB (DSB)-independent [48] . Previous reports that cells lacking RNase HI and DSE-repair enzyme RecBCD are inviable suggested that RNase H-defective cells might have more DSEs than wild-type [35] , [49] . The results presented here support this interpretation with more direct data (for example, Figs 5 and 8 ) and add to it that the R-loops are transcriptional ( Figs 1 , 2 , 3 , 4 ) and that DSE generation by R-loops additionally requires a ssDNA nick ( Figs 7 and 8 ), thus providing strong support for the specific mechanism shown in Fig. 1a–f . R-loops are identified here as the earliest known molecular intermediate in stress-induced amplification and point mutation in E. coli . R-loops might also underlie other instances of DSE formation that instigates genomic instability in stressed cells in which replication is likely to be inhibited. For example, collapse of R-loop-generated forks might underlie the DSEs that drive bile-induced resistance mutagenesis in pathogenic Salmonella [6] , DSEs that create genetic diversity in biofilms of pathogenic Pseudomonas [4] , genomic instability leading to cancer initiation in cells of non-proliferating tissues, and cancer and pathogen resistance to growth-arresting chemotherapies. DSBs/DSEs of unknown origin are hypothesized to underlie mutation hotspots in cancer genomes [50] , [51] , as demonstrated in E. coli [25] , and might similarly be instigated by the R-loop-generated fork-collapse-at-nick mechanism shown here. R-loops are also implicated in replication initiation in ColE1 plasmids [52] , mouse mitochondrial replication [53] and class-switch recombination and somatic hypermutation in the mammalian immune system (reviewed by Chaudhuri and Alt [54] ). R-loops are associated with hyper-recombination, genomic instability and DSBs from bacteria to yeast and human (reviewed by Li and Manley [55] ). R-loops underlie breakage at common fragile sites in human [56] . Some of these instances of breakage require replication as well as transcription [18] , [56] , and so might also result from R-loop-generated fork collapse at nicks. Transcription was implicated previously in DSB-dependent mutagenesis in E. coli in that a strain with a partially-defective NusA transcription anti-termination factor shows reduced SIM, and might do so via reduced interactions with DinB error-prone DNA polymerase [57] . Our data suggest a possible alternative explanation that could unite their data and ours. R-loops form preferentially at particular DNA sequences, hypothesized to have special structural features [35] . When NusA is functional, some transcripts will be longer (anti-terminated). Perhaps, in the presence of functional NusA, a transcript that would otherwise not reach a site prone to stable R-loop formation reaches such a site, such that R-loops are formed or stabilized, promoting SIM. This model and others remain to be tested. The association of transcriptional R-loops with DSEs opens the possibility that in addition to being targeted preferentially to times of stress, by their coupling to the stress responses [7] , [9] and see Al Mamun et al . [30] ), stress-induced point mutation and amplification could be targeted preferentially to regions of active transcription. DSE-dependent point mutagenesis occurs in strong hotpots maximally within two and up to 60 kb from a DSE [25] . This means that transcription-produced DSEs would be expected to cause hotspots of mutations near sites of transcription. The suggestion that DSBs cause the hotspots observed in cancer genomes and chemically damaged yeast cells [50] , [51] suggests the possibility of transcriptional/R-loop targeting of mutations also in cancer genomes. Transcription also promotes local SIM in starving B. subtilis cells, though apparently independently of DSEs and recombination [58] . In stressed cells, actively transcribed regions are likely to harbour genes whose products counter the stress. Thus, stress-induced point mutations and genome rearrangements might occur preferentially where they are most likely to affect phenotypes immediately, including advantageously. Both regulation of mutagenesis in time, by stress responses, and in genomic space, by linkage with transcription and DSEs, could enhance the ability to evolve during stress for small populations in which mutation supply is limiting. Strains Strains and plasmids used in this study are listed in Supplementary Table S3 and are isogenic with SMR4562, an independent construction of FC40 (ref. 29 ). FC40/SMR4562 carry a +1 frameshift mutation in a lacI–lacZ fusion gene in F′ plasmid F′128. FC29 (ref. 29 ) is an F′-carrying non-revertible lac deletion strain that is used to scavenge extraneous carbon sources from minimal lactose plates. SMR5383, an ampicillin-resistant ara − scavenger derived from FC29, was used in experiments involving pBAD constructs or plasmids. Δ mfd and Δ rnhA alleles were introduced into strains by P1 transduction. SIM experiments Lac - E. coli were grown in minimal glycerol medium to prolonged stationary phase, plated onto minimal lactose solid medium and incubated for 7 days at 37 °C [22] . The Lac + colonies that arise each day are counted and marked. They have acquired either a compensatory-frameshift (‘point’) mutation, or amplification of the leaky lac allele to 20 or more copies, which allows growth without a reversion mutation [36] . Amplification of lac is unstable under nonselective conditions, so lac- amplified clones can be identified by plating cells from Lac + colonies onto nonselective medium containing 5-bromo-4-chloro-3-indoyl-β- D -galactoside (X-gal) on which lac- amplified isolates show a sectored appearance. In spectinomycin-pulse experiments, 100 μg ml −1 spectinomycin was added 3 h before plating and then washed from cells before plating on minimal lactose medium. All experiments were performed ≥3 times, and repeat experiments gave consistent results. Representative graphs were chosen for illustration and summaries of mutation rate data from multiple experiments (mutations per cell per day) are given in the text. In experiments with plasmid pBAD18-rnhA overproducing RNase HI, 100 μg ml −1 ampicillin was added to the minimal lactose plates to maintain the plasmid. The arabinose is not catabolized (the cells still starve) because the cells are ara − . Plugs of agar from these plates were taken with capillary pipettes periodically during the experiment, resuspended and plated for colony-forming units on plates with and without ampicillin to verify that cells retained the plasmid. No significant plasmid loss was observed. To produce RNase HI, 5 × 10 −8 (w/v) arabinose was added to the minimal lactose plates. This concentration was chosen because we found that higher concentrations caused inhibition of growth. The same concentrations of ampicillin and arabinose were used in experiments with I- Sce I and overproduction of RNase HI. The arabinose induces production of both RNase HI and I- Sce I. In I- Sce I experiments, the number of ampicillin-resistant cells carrying the plasmid was similar for the control and RNase HI-producing plasmids (0.77±0.09 versus 0.70±0.16, respectively, in cells recovered from lactose plates after 1 day, mean±s.e.m. ), and did not change significantly during the experiment. The proportion of cells showing resistance to arabinose (indicating loss of the I- Sce I cut site [21] ) was not different between the DSB-inducing strains with and without the RNase HI plasmid (0.19±0.02 versus 0.22±0.02, respectively, in the experiment shown). For experiments in Fig. 6 , Gam was induced by doxycycline at 100 ng ml −1 applied for 48 h from early stationary phase. Inducible Gam and GAMGFP of phage Mu Details of construction and validation of the chromosomally expressed inducible Gam and GamGFP will be published separately. In brief, the Eco RI fragment of the bacteriophage Mu gam gene from plasmid pJA21 [59] was sub-cloned downstream from the P N25 tetO promoter [60] , a promoter that can be induced by tetracycline or doxycycline, in cells carrying P N25 tetR , encoding a constitutive Tet repressor, which represses transcription from P N25 tetO in non-inducing conditions [60] . P N25 tetOgam was placed in the E. coli chromosome. Similarly, the gam-gfp fusion gene, to be described elsewhere, was placed downstream of the P N25 tetO . For experiments in Fig. 8 , production of GamGFP was induced in log-phase with 100 ng ml −1 doxycycline for 3 h. Cells were concentrated and placed on slides and photographed in bright field and phase contrast. At least ten fields of ~10–100 cells were counted for each sample. Samples were scored blindly as focus-containing or not. How to cite this article: Wimberly, H. et al . R-loops and nicks initiate DNA breakage and genome instability in non-growing Escherichia coli . Nat. Commun. 4:2115 doi: 10.1038/ncomms3115 (2013).